Magnetocaloric effects in a freestanding and flexible graphene-based superlattice synthesized with a spatially confined reaction Superlattices have attracted great interest because of their tailorable electronic properties at the interface. However, the lack of an efficient and low-cost synthetic method represents a huge challenge to implement superlattices into practical applications. Herein, we report a space-confined nanoreactor strategy to synthesize flexible freestanding graphene-based superlattice nanosheets, which consist of alternately intercalated monolayered metal-oxide frameworks and graphene. Taking vanadium oxide as an example, clear-cut evidences in extended X-ray absorption fine structure, high-resolution transmission electron microscopy and infrared spectra have confirmed that the vanadium oxide frameworks in the superlattice nanosheets show high symmetry derived from the space-confinement and electron-donor effect of graphene layers, which enable the superlattice nanosheets to show emerging magnetocaloric effect. Undoubtedly, this freestanding and flexible superlattice synthesized from a low-cost and scalable method avoids complex transferring processes from growth substrates for final applications and thus should be beneficial to a wide variety of functionalized devices. Superlattices have been the subject of active research in the past two decades because of their fascinating physical phenomena arising from new electronic states at the interface [1] , which opens exciting opportunities to design new materials with novel properties [2] , [3] . Since the first experimental superlattice growth by molecular beam epitaxy [4] , a spectacular series of advances has been accomplished in areas such as the discovery of high-temperature superconductors [5] , integer and fractional quantum Hall effect [6] , [7] , giant and colossal magnetoresistance [8] , [9] and topological insulators [10] , [11] . However, the conventional superlattice-fabrication strategies are usually based on pulsed laser deposition or molecular beam epitaxy, which are complex and expensive as well as involve difficulty in the transferring process from the growth substrate for final application [12] . In fact, the lack of an efficient and low-cost synthetic method represents a huge challenge to implement superlattices in practical applications, which inspires us to further pursue the low-cost and scalable bottom-up techniques for the synthesis of superlattices. Graphene, consisting of stacked sheets (<10) of two-dimensional sp 2 -hybridized carbon atoms arranged in six-membered rings, has generated enormous interest in the past years because of its prominent intrinsic properties and great potential in various applications [13] , [14] . The unique electronic structure of graphene endows its extraordinary ambipolar electronic property, which implies that graphene can serve as an electron donor or acceptor to continuously tune the holes and electrons when combined with other substances. In this sense, graphene is a good matrix for hybrid materials and in particular graphene-based superlattices [15] , [16] , [17] , [18] , [19] , which are envisaged to synergistically offer tremendous opportunities for improving and expanding applications. On the other hand, as is well known, few-layered graphene is an intermediate state between graphite and monolayered graphene, which shows superiority over graphite and monolayered graphene for growing graphene-based superlattice, for the interlayer spacing of few-layered graphene is remarkably larger than that of graphite. At the same time, the graphene nanosheets could be better stacked compared with monolayered graphene. Therefore, few-layered graphene is a perfect material for growing such graphene-based superlattice. Owing to the discovery of many distinctive physical properties, such as superconduction [20] , [21] , superionic conduction [22] , [23] , giant magnetocaloric effect [24] , [25] , optical storage [26] and so on [27] , the subject of phase transition in solid materials has grown continuously and enormously for centuries, forming not only the basis of materials technology but also the central issue of solid-state chemistry. VO 2 is a well-known prototype material to understand the electronic structure and related physical properties during phase transitions [28] . For example, in the rutile VO 2 (R), the isometric V–V bond (2.88 Å) results in itinerant 3 d electrons in the overlapping V 3 d orbitals, leading to an electrically conducting state. Meanwhile, in the monoclinic VO 2 (M), the V–V bond splits into alternately altered bond lengths of 2.62 and 3.16 Å; thus, the outer V 3 d electrons are localized, which results in an electrically insulating state. As temperature varies, a fully reversible structural phase transition process associated with optical, electric and magnetic property changes takes place between these two phases of VO 2 . Although VO 2 (M/R) has been regarded as a thermodynamically stable phase, it needs to overcome a high reaction barrier to form this phase in a solution reaction system. As a result, a metastable phase with shear structure consisting of vertex and edge sharing of deformed VO 6 octahedra, VO 2 (B), is regarded as the most common phase obtained from solution reactions [29] , which has been used as the exclusive precursor for obtaining VO 2 (M/R) through solid-state transformation, even though this transformation usually requires the rigid synergic effects of high-temperature post treatment, inert-gas atmosphere with precisely controlled flow and long synthesis time [30] . Recently, our group reported that the injection of electrons into the V–O systems by adventitious hydrogen can lead to an enhancement of the e–e correlation effects and strengthening of the electronic orbital overlap of the infinite V–V chains, which results in the stabilization of high-temperature-phase metallic VO 2 (R) at room temperature [31] . These facts suggest that the introduction of structural lattice perturbation by an additional substance would simultaneously activate the spin, charge and/or orbital of a material, and would provide an effective way to modulate its electronic structure, resulting in a controllable electronic structure and its related physical properties. Here we report a space-confined method to synthesize graphene-based superlattices, in which the graphene layers provide not only a space-confined nanoreactor to direct the growth of monolayered metal oxide frameworks in a two-dimensional manner, but also serve as an electron donor to reduce the formation energy for highly symmetrical metal-oxide frameworks. The electron transfer and stress field at the interface of the superlattice lead to the structural rearrangements of the metal-oxide frameworks, which endow the superlattice nanosheets more fascinating physicochemical properties. Taking vanadium oxide as an example, we experimentally obtain the freestanding and flexible vanadium oxide/graphene superlattice nanosheets, which show significantly enhanced magnetocaloric effect compared to that observed in the VO 2 (M)–VO 2 (R) phase transition. Likewise, these superlattice nanosheets also show smart switching behaviour in electrical conductivity and near-IR optical as well as magnetic properties, which are very attractive for intelligent devices such as temperature sensors. Structural identification These graphene-based superlattices were synthesized in a space-confined nanoreactor formed by the interlayers of reduced graphene oxides (RGO) (as seen in Fig. 1 ). As is well known, RGO nanosheets usually possess some oxygen-containing groups, such as hydroxyl groups and carboxylic acid groups, which make the RGO negatively charged after dispersing in water. Meanwhile, the VO(acac) 2 hydrolyse to the positively charged species of [VO(H 2 O) 5 ] 2+ in water, which can intercalate into the interlayers of negatively charged RGO nanosheets through the electrostatic attraction effect. Under the following solvothermal reaction condition, the homogenously intercalated [VO(H 2 O) 5 ] 2+ condenses to VO 6 octahedra in the RGO’s interlayers formed space-confined nanoreactor, which yields the homogenously distributed superlattice. During the condensation polymerization process, the oxygen-containing groups on RGO develop to act as bridging oxygen between the graphene layer and the V–O framework, through which the electron transfer process occurs between the graphene layer and the V–O framework. As demonstrated in our previous report [29] , the VO(acac) 2 first hydrolyses to [VO(H 2 O) 5 ] 2+ and then condenses to VO 6 octahedra, and the vertex and edge sharing of this VO 6 octahedra usually form VO 2 (B) in an open solution reaction system, which is confirmed by a parallel experiment where other experimental conditions are kept the same except for absence of RGO (see Supplementary Fig. 1 ). However, in this space-confined nanoreactor strategy, the graphene layers could provide a space-confined nanoreactor to avoid the fast aggregation of VO 6 octahedra and direct the VO 6 octahedra to connect with each other in a two-dimensional manner, forming a monolayered V–O framework similar to monolayered VO 2 (B), with some structural deformation, which is also observed in exfoliated VO 2 (B) [32] . Furthermore, the V–O framework could accept electrons from graphene to reduce the formation energy for obtaining a high symmetry. As expected, X-ray absorption fine structure spectroscopy, a powerful element-specific tool to study the local atomic arrangements and electronic structures of condensed matters, provides evidence on the formation of highly symmetric V–O frameworks in the superlattice nanosheets. Extended X-ray absorption fine structure (EXAFS) spectroscopy is the measurement of the x-ray absorption coefficient of a material as a function of energy, typically in a 500-1000 eV range beginning before the absorption edge of an element in the sample. It is a useful tool for the investigation of local bond lengths in the environment of a given element. The k 3 χ ( k ) EXAFS oscillation curves shown in Fig. 2a reveal remarkable differences between the V–O framework of the superlattice nanosheets and VO 2 (B) in the k -region, implying the different local atomic arrangement. These differences are further illustrated by the Fourier transformed (FT) k 3 χ ( k ) functions in R -space shown in Fig. 2b . The intensities of the nearest V–O and V–V coordination shells of the superlattice nanosheets are reduced compared with VO 2 (B) because the degree of order in the V–O framework in the superlattice nanosheets was decreased. The schematic structure model of the intercalated V–O framework is presented in Fig. 2c,d , which is obtained from the quantitative fitting results of the V–O bonds (see Supplementary Fig. 2 ). Compared with VO 2 (B), the V–O framework in the superlattice nanosheets exhibits a more symmetric structure. The highly symmetrical V–O framework in superlattice nanosheets shows a zigzag V–V chain with an isometric bond length of about 2.77 Å, which corresponds closely to the value of linear V–V chains with an isometric bond length of 2.88 Å in VO 2 (R) [33] ; thereby both of the V–V chains in the superlattice nanosheets and VO 2 (R) are derived from the edge sharing of the adjacent VO 6 octahedron. Except for a more symmetric structure, the V–O framework of the superlattice nanosheets possesses an expanded structure along the intercalation direction. This means that the average length of the V–O bonds along the intercalation direction is elongated compared with VO 2 (B), which may be the result of the electron transfer from the graphene layer to the V–O framework layer. This electron transfer is confirmed by Raman spectra. Figure 2e shows the typical Raman spectra recorded for RGO and the obtained superlattice samples, which yield D bands at 1346 and 1378, cm −1 , respectively. 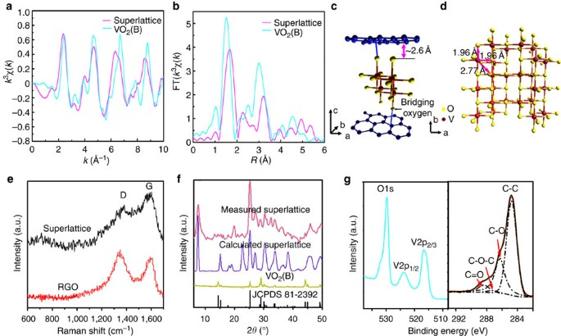Figure 2: Atomic arrangements and structural characterization of the superlattice nanosheets. (a) VK-edge extended XAFS oscillation functionk3χ(k) and (b) Fourier transforms ofk3χ(k) for the V–O framework in superlattice nanosheets and VO2(B), respectively. (c,d) Representative atomic models of superlattice nanosheets extracted from the quantitative fitting results of the V–O and V–V bonds. (e) The Raman spectra for the obtained superlattice and starting RGO, respectively. (f) Experimental XRD patterns of the superlattice nanosheets and VO2(B). The standard pattern of VO2(B) in JCPDS card no. 81-2392 and the calculated XRD pattern of the constructed model structure of superlattice nanosheets are also shown. (g) The XPS spectra of the obtained superlattice. Compared to RGO, the D band of the superlattice shows a clear Raman peak shift towards high frequency and intensity reduction, which demonstrates the electron transfer from the graphene layer to the V–O framework layer. (A detailed explanation is provided in Supplementary Fig. 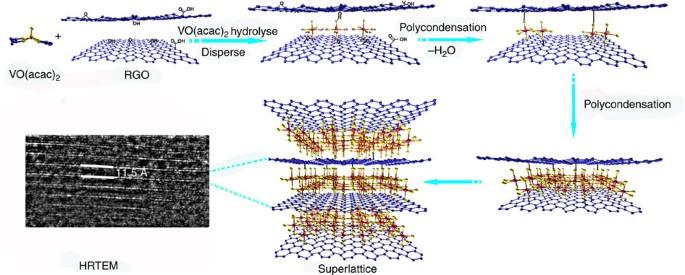3 and Supplementary Note 1 .) Figure 1: Schematic representation of the formation mechanism for the superlattice through space-confined nanoreactor strategy. VO(acac)2is firstly hydrolysed to yield [VO(H2O)5]2+, then intercalated into the interlayers of RGO nanosheets. The intercalated [VO(H2O)5]2+condenses to VO6octahedra in the RGO interlayers formed space-confined nanoreactor. Finally the VO6octahedra further condenses to yield vanadium oxide nanosheets in the interlayers of RGO nanosheets, resulting in the formation of the superlattice. Figure 1: Schematic representation of the formation mechanism for the superlattice through space-confined nanoreactor strategy. VO(acac) 2 is firstly hydrolysed to yield [VO(H 2 O) 5 ] 2+ , then intercalated into the interlayers of RGO nanosheets. The intercalated [VO(H 2 O) 5 ] 2+ condenses to VO 6 octahedra in the RGO interlayers formed space-confined nanoreactor. Finally the VO 6 octahedra further condenses to yield vanadium oxide nanosheets in the interlayers of RGO nanosheets, resulting in the formation of the superlattice. Full size image Figure 2: Atomic arrangements and structural characterization of the superlattice nanosheets. ( a ) V K -edge extended XAFS oscillation function k 3 χ ( k ) and ( b ) Fourier transforms of k 3 χ ( k ) for the V–O framework in superlattice nanosheets and VO 2 (B), respectively. ( c , d ) Representative atomic models of superlattice nanosheets extracted from the quantitative fitting results of the V–O and V–V bonds. ( e ) The Raman spectra for the obtained superlattice and starting RGO, respectively. ( f ) Experimental XRD patterns of the superlattice nanosheets and VO 2 (B). The standard pattern of VO 2 (B) in JCPDS card no. 81-2392 and the calculated XRD pattern of the constructed model structure of superlattice nanosheets are also shown. ( g ) The XPS spectra of the obtained superlattice. Full size image The superlattice structure has been verified by XRD as shown in Fig. 2 . As seen from the XRD patterns, compared to that of the starting graphene oxide (GO) and RGO (see Supplementary Fig. 4 ), a newly arising d -spacing at d =11.5 Å appears in the superlattice nanosheets, implying a new interlayer distance. The measured XRD pattern of the superlattice nanosheets matches well with the calculated XRD pattern of the constructed model structure with alternately intercalated V–O frameworks and graphene layers.The transmission electron microscope (TEM) image and the selected area electron diffraction (SAED) patterns were recorded to further confirm the superlattice structure. As seen from Fig. 3a , the corresponding TEM image confirms the two-dimensional (2D) morphology of the as-obtained superlattice nanosheets. Meanwhile, the folded cross-section edge confirms the flexibility of our superlattice nanosheets, which is different from that of the synthetic superlattice obtained by pulsed laser deposition or molecular beam epitaxy, implying a more practical use in applications, especially in the flexible functionalized devices. The high-resolution TEM (HRTEM) image and SAED pattern of the cross-section edge shown in Fig. 3b indicate the existence of a distinctive superlattice structure that consists of 11.5 Å periodic slabs along the [001] direction. The periodicity of 11.5 Å is approximately the sum of the layer spacings of vanadium oxide and graphene, agreeing well with the XRD results and suggesting that the monolayered V–O frameworks alternately intercalate into the adjacent graphene layers. A HRTEM image of the basal plane is shown in Fig. 3c , in which the interplanar spacings were measured to be 1.99 and 1.40 Å according to the periodic pattern of the lattice fringes, matching up with the plane spacings of the fitted V–O framework by EXAFS (inset in Fig. 3c ), respectively. The corresponding SAED pattern of the basal plane (as seen in Fig. 3d ) displays a strong spot pattern associated with elongated satellite spots, indicating that the graphene layers are distorted in the V–O framework layers, which has been widely recognized in superlattice intercalate systems of a Bragg signature of a modulated structure [34] , [35] . The uniformity of this obtained superlattice is subjected to detailed discussion in Supplementary Fig. 4 and Supplementary Note 2 . X-ray photoelectron spectroscopy (XPS) ( Fig. 2g ) was also done to ascertain the composition of the superlattice. The two peaks at 516.5 and 523.7 eV can be attributed to V2p 2/3 and V2p 1/2 (ref. 32 ), respectively The deconvoluted C-1s XPS spectrum shows the four peaks at 284.8, 286.3, 287.2 and 288.3 eV, due to C–C, C–O, C–O–C and C=O bonding, respectively [36] . 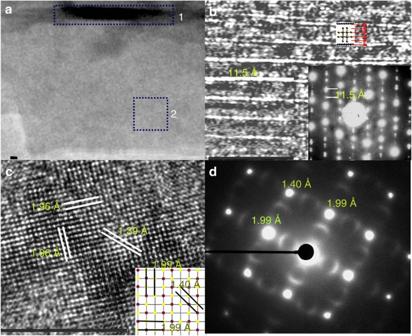Figure 3: TEM and HRTEM images of the superlattice nanosheets. (a) Low-magnification TEM image confirms the two-dimensional (2D) morphology and flexibility of our as-obtained superlattice nanosheets, (b) HRTEM image of the cross-section edge of the superlattice nanosheets as highlighted by dotted box 1 in (a). The inset of (b) shows the corresponding SAED pattern of the cross-section edge. (c) HRTEM image of the basal plane of the superlattice nanosheets as highlighted by dotted box 2 in (a). The inset of (c) shows the interplanar spacing obtained from the structure models. (d) Corresponding SAED pattern of the basal plane. Scale bar, 5 nm. Figure 3: TEM and HRTEM images of the superlattice nanosheets. ( a ) Low-magnification TEM image confirms the two-dimensional (2D) morphology and flexibility of our as-obtained superlattice nanosheets, ( b ) HRTEM image of the cross-section edge of the superlattice nanosheets as highlighted by dotted box 1 in ( a ). The inset of ( b ) shows the corresponding SAED pattern of the cross-section edge. ( c ) HRTEM image of the basal plane of the superlattice nanosheets as highlighted by dotted box 2 in ( a ). The inset of ( c ) shows the interplanar spacing obtained from the structure models. ( d ) Corresponding SAED pattern of the basal plane. Scale bar, 5 nm. Full size image Emergence of the phase transition and its characterization As aforementioned, due to the space-confinement effect, the V–O frameworks in the superlattice nanosheets show high symmetry with an isometric V–V bond length of about 2.77 Å, similar to the VO 2 (R), which allows us to predict that it will show similar properties to that of the VO 2 (R). The apparent endothermic and exothermal peaks in the differential scanning calorimetry (DSC) curves (as shown in Fig. 4a ) undoubtedly indicate reversible first-order phase transition in our superlattice nanosheets. FT infrared (FTIR) spectroscopy was also used to further confirm the phase transition in the superlattice nanosheets because the vibration frequencies of chemical bonds vary with the atoms’ geometric arrangement, providing a ‘fingerprint’ information in a given molecular structure [37] . As shown in Fig. 4b,c , the high-temperature FTIR spectra show absorbing peaks at 560, 926 and 1,003 cm −1 , which can be indexed to the edge-sharing V–O stretching vibration, V–O–V bending vibration and V=O stretching vibration in the V–O framework, respectively, while the peaks at 1,109, 1,400 and 1,645 cm −1 can be indexed to vibrations of C-O, –OH, and –C=O in the graphene layers. 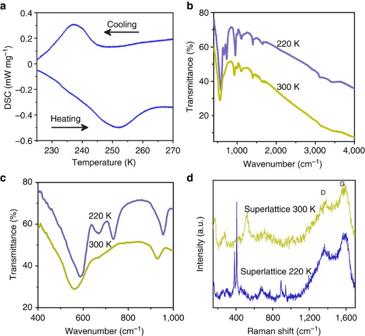Figure 4: Optical and electrical properties of the superlattice nanosheets. (a) DSC thermogram, (b) temperature-dependent FTIR spectra indicate that the superlattice nanosheets experience a first-order phase transition as temperature varies. (c) The magnified FTIR spectra. The temperature-dependent FTIR spectra also imply the optical switching of the superlattice nanosheets in middle-wavelength IR regions. (d) Temperature-dependent Raman spectra of the obtained superlattice. Evident difference in the absorbing peaks arises at about 560 and 926 cm −1 corresponding to a blue shift of Δ =26 and 30 cm −1 , respectively, as the temperature decreased across the transition point, implying the symmetry breakdown of the V–O framework below the transition temperature, which is analogous to the change of IR spectra during the phase transition of VO 2 (M) and VO 2 (R) at around 340 K. Figure 4: Optical and electrical properties of the superlattice nanosheets. ( a ) DSC thermogram, ( b ) temperature-dependent FTIR spectra indicate that the superlattice nanosheets experience a first-order phase transition as temperature varies. ( c ) The magnified FTIR spectra. The temperature-dependent FTIR spectra also imply the optical switching of the superlattice nanosheets in middle-wavelength IR regions. ( d ) Temperature-dependent Raman spectra of the obtained superlattice. Full size image Next, we employed Raman spectroscopy to confirm the phase transition of the superlattice, since rotational and vibrational information specific to the chemical bonds and symmetry of molecules could be inferred from the shifted frequencies. As seen in Fig. 4d , the Raman spectra of the superlattice show distinct difference between the high-temperature phase and low-temperature phase. Except for the peaks of graphene (1,300–1,600 cm −1 ), most of the Raman peaks ascribed to the low-temperature phase disappeared as temperature increased to room temperature. The distinctly dwindled numbers of Raman shift peaks in the high-temperature phase indicate that the V–O framework in the superlattice at high temperature is of higher symmetry. It is noteworthy that the IR transmittance is connected through metallic free electrons, the so-called free electrons in metallic materials are responsible for electrical conductivity and their excitation energies match with the light energies of the IR wavelength; thus the IR light is reflected off or absorbed rather than transmitted in a metallic (or narrow gap semiconductor) material. On the other hand, in isolating materials the excitation energies are much larger than the energies of the IR light and thus the IR spectrum is transmitted. The temperature-dependent resistivity curve in Supplementary Fig. 5 leads us to the conclusion that the superlattice nanosheets undergo a first-order transition at about 252 K from an insulating to a narrow-gap semiconductor phase, accompanied by remarkable IR optical switch as temperature increases. Besides, the magnetism of the space-confined synthesized superlattice nanosheets also shows emergent behaviour: an abrupt change in the magnetic susceptibility ( Fig. 5a ) was observed as the temperature decreased, which is similar to the effect in VO 2 (R) (ref. 38 ). Considering that the highly symmetric V–O framework in the superlattice nanosheets has zigzag V–V chains with an isometric bond length of about 2.77 Å, analogous to the linear V–V chain in VO 2 (R) by edge sharing of the regular VO 6 octahedron, a similar rearrangement of V–V chains may take place in the superlattice nanosheets, and should be responsible for the observed change in magnetism. For comparison, the M–T curve of VO 2 (B) synthesized from the same raw materials in the open solution reaction system was also measured, and the result ( Fig. 5a ) clearly showed no abrupt change in the magnetic susceptibility of VO 2 (B), consistent with the M–T curve reported previously [39] . This result indicates that the atomic arrangement of the V–O framework in the superlattice nanosheets is indeed different from that of VO 2 (B), presumably because of the space-confinement effect of graphene. 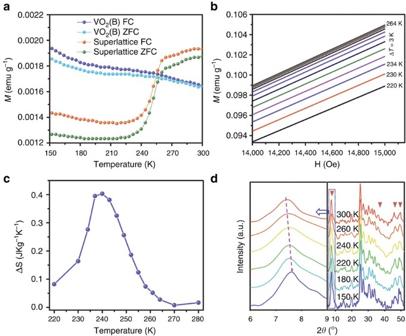Figure 5: Magnetic properties of the superlattice nanosheets. (a) Temperature-dependent ZFC and FC magnetization in an applied field of 100 Oe for the superlattice nanosheets and VO2(B). (b) The field-dependent magnetization plots at indicated temperatures. (c) Magnetic entropy change ΔSof the superlattice nanosheets. (d) Temperature-dependent XRD patterns for the superlattice nanosheets. Figure 5: Magnetic properties of the superlattice nanosheets. ( a ) Temperature-dependent ZFC and FC magnetization in an applied field of 100 Oe for the superlattice nanosheets and VO 2 (B). ( b ) The field-dependent magnetization plots at indicated temperatures. ( c ) Magnetic entropy change Δ S of the superlattice nanosheets. ( d ) Temperature-dependent XRD patterns for the superlattice nanosheets. Full size image The magnetocaloric effect of the superlattice Generally, a magnetic substance shows magnetocaloric effect in a reversible magnetic susceptibility change experience through adiabatic magnetization or demagnetization, which has been used as an environmentally friendly and highly efficient cooling technology to replace conventional gas compression refrigeration during the past decades [40] , [41] , [42] , [43] , [44] . In our present work, the field dependence of magnetization for the as-obtained superlattice nanosheets was measured up to 1.5 T in the temperature range from 220 to 300 K, and the representative M–H curves are presented in Fig. 5b and Supplementary Fig. 6 . The magnetization increases progressively with increasing temperature, presenting a step-like behaviour in the temperature range covering the phase transition. This step-like behaviour in the M–H curve provides direct information on the magnetocaloric effect because the magnetocaloric effect is related to the rearrangement of the magnetic moment under a magnetic field caused by either pure magnetic or lattice transformation. The magnetic entropy change can be calculated from the M–H data on the basis of the Maxwell relation equation [37] : The temperature dependence of Δ S was calculated and plotted in Fig. 5c . The maximum value of Δ S is about 0.4 J kg −1 K −1 , which is remarkably larger than that of the VO 2 (M)–VO 2 (R) phase transition-driven magnetocaloric effect [38] . As is known, the rapid change of magnetization would cause a large magnetic entropy change, resulting in larger magnetocaloric effect. The orientation of sharing V d -orbit electrons in a V–V chain should be responsible for the magnetic transformation from magnetic moment disordering to ordering, which means a single-domain structure could be expected to benefit from the rapid magnetization change. In our single-crystalline superlattice nanosheets, the V–O frameworks are confined to the interlayer of multilayered graphene, and all of the V–O frameworks are parallel, which should form the single-domain structure to realize the rapid magnetization change resulting in the larger magnetocaloric effect. On the other hand, the structural transition-driven magnetocaloric materials usually show strong coupling between crystallographic structure and magnetism; thus, any induced changes in the lattice entropies during the phase transition should also contribute to the ultimate performance of the magnetocaloric effect [45] . In fact, recent reports have discovered that the strain-mediated feedback from substrates near the first-order phase transition can strongly enhance the total magnetocaloric effect [46] , [47] . In our present work, as aforementioned, the V–O frameworks are confined to the interlayer of the multilayered graphene; thus, it is reasonable to believe that extrinsic strain feedback from the graphene layers to the intercalated V–O frameworks should exist, which has been verified through the temperature-dependent XRD. As seen from Fig. 5d , with decreasing temperature, the shift of the low-angle diffraction peak towards higher 2 θ values indicates that the distance between two graphene layers is gradually shortened. This means that the graphene layers exert extrinsic strain on the V–O frameworks, resulting in an enhanced Δ S value compared to that of our previously reported VO 2 (M)–VO 2 (R) phase transition-driven magnetocaloric effect. In summary, the space-confined strategy within the interlayers of multilayered graphene enables the synthesis of freestanding and flexible superlattice nanosheets with special atomic configuration of the component to realize emerging physicochemical properties. In this approach, taking VO 2 as an example, the graphene layers not only provide a space-confined nanoreactor to avoid the fast aggregation of VO 6 octahedra and direct the VO 6 octahedra to connect each other in a two-dimensional manner, but also serve as an electron donor to reduce the formation energy to obtain highly symmetrical V–O frameworks. These highly symmetrical V–O frameworks endow the obtained superlattice nanosheets emerging magnetocaloric effect compared to the VO 2 (B) sample obtained from the same raw materials in the open solution-reaction system. Owing to the two-dimensional single-domain structure of the V–O frameworks and extrinsic strain exerted by graphene layers, the Δ S value of the superlattice nanosheets was significantly enhanced compared to that observed in the VO 2 (M)–VO 2 (R) phase transition. These flexible freestanding superlattice nanosheets synthesized from a low-cost and scalable method avoid the complex transferring process from growth substrates, as required in conventional synthesizing strategies, and thus can be adapted to a large variety of applications in functionalized devices. Synthesis of grapheme Firstly, GO was prepared via a modified Hummer’s method. After removing the salts and acids, the GO was ultrasonically treated in water for over 1 h until it became clear without visible particles to form GO collosol. Then the collosol was transferred into a 250-ml round-bottom flask, followed by addition of 0.031 ml hydrazine hydrate (85%) and 0.784 ml ammonia solution (25%) into the flask under stirring. Then the solution was heated in an oil bath to 100 °C using a water-cooled condenser for 24 h. Finally, the as-obtained RGO black collosol was cooled to room temperature for further intercalation. Synthesis of superlattice nanosheets The RGO precursor was exfoliated under ultrasonic treatment for several hours to obtain small and thin RGO pieces, and an RGO solution was obtained: 0.18 mmol VO(acac) 2 and 0.8 ml H 2 O 2 were dissolved in 30 ml acetone, then 4 ml of the RGO solution was added, subjected to magnetic stirring for several minutes and then ultrasonicated for about half an hour to intercalate the vanadium source homogenously into the interlayer of adjacent RGO nanosheets. Then the well-distributed suspension was transferred into a 40 ml stainless Teflon-lined autoclave followed by solvothermal process at 180 °C for 24 h. Afterwards the system was cooled to room temperature in air. The product was collected by centrifugation at 10,000 r.p.m. for 2 min, washed with distilled water and ethanol, and dried in vacuum at 60 °C for 8 h. For comparison, a product without graphene was prepared according to the above-mentioned process. Characterization The phase structure of the product was characterized by X-ray powder diffraction (XRD) using a Philips X’Pert Pro Super diffractometer with a Cu K α radiation source ( λ =1.54178 Å). Field emission scanning electron microscopy (FESEM) images were obtained using a JEOL JSM-6700F scanning electron microscope. The TEM, HRTEM images and SAED analyses were captured by a JEOL JEM-ARF200F atomic resolution analytical microscope. Raman spectrum was performed on a SPEX 1403 spectrometer equipped with an Ar + laser at an excitation wavelength of 514.5 nm. The XPS spectrum was recorded by a VGESCALAB MK|X-ray photoelectron spectrometer with an Al K α . exciting source. The magnetization was characterized by a superconducting quantum interference device (SQUID, quantum design MPMS XL-7) magnetometer. The XAFS spectra of the superlattice nanosheets were measured at the U7C beamline of the National Synchrotron Radiation Laboratory. How to cite this article: Zhu, H. et al . Magnetocaloric effects in a freestanding and flexible graphene-based superlattice synthesized with a spatially confined reaction. Nat. Commun. 5:3960 doi: 10.1038/ncomms4960 (2014).